Distinct molecular pathways mediate Mycn and Myc-regulated miR-17-92 microRNA action in Feingold syndrome mouse models 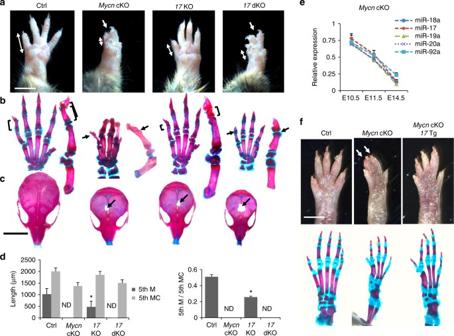Fig. 1 Generation of mouse models of Feingold syndrome.aForelimbs of wildtype control (Ctrl),MycnKnockout (Prx1-Cre:Mycnfl/fl,MycncKO),Mir17-92knockout (Prx1-Cre:Mir17-92fl/fl,17KO), andMir17-92andMir106b-25doubly conditional knockout (Prx1-Cre:Mir17-92fl/fl:Mir106b-25−/−,17dKO) mice at postnatal day (P) 16.17KO mutants exhibit mild brachydactyly in the fifth digit (double-headed arrows). Cutaneous syndactyly (arrows) and severe brachydactyly are presented in17dKO andMycncKO mice. Scale bar, 0.5 cm.bAlizarin red and alcian blue staining of the forelimb and magnified views of the fifth digit of corresponding mice ina.17KO mutants show shortening of the middle phalanx (M) (brackets) of the fifth digit.17dKO andMycncKO mutants show severe brachymesophalangy and the absence of the middle phalanx of the fifth digit (arrows).cAlizarin red and alcian blue staining of the skull of corresponding mice ina.MycncKO,17 KO, and17dKO mice show microcephaly and a frontal bone ossification defect (arrows). Scale bar, 1 cm.dQuantification of the length of the fifth M and fifth metacarpal bone (5th MC) and the ratio of 5th M to 5th MC. Values are expressed as mean ± SE (n= 5 in each group, *p< 0.001 vs. Ctrl). ND, not detected.eRelative expression of five miRNAs encoded in the Mir17-92 gene in limb bud mesenchymal cells isolated fromMycncKO embryos at embryonic day 14.5. (relative to control littermate samples,n= 5 each group, *<0.001 vs. Ctrl at every time point).fHindlimbs of wildtype Ctrl,MycncKO, andMycnKnockout overexpressingMir17-92(Prx1-Cre:Mycnfl/fl:Mir17-92Tg, MycncKO:17Tg) (upper panels) and alizarin red and alcian blue staining of the hindlimbs of corresponding genotypes (bottom panels).Mir17-92overexpression partially rescues the skeletal defects ofMycncKO mutants. Cutaneous syndactyly (white arrows) and shortening of the fifth digit inMycncKO mutants are rescued by overexpression ofMir17-92whereas fused fourth and fifth metatarsal bones still remain (bottom panels). Scale bar, 0.5 cm Feingold syndrome is a skeletal dysplasia caused by loss-of-function mutations of either MYCN (type 1) or MIR17HG that encodes miR-17-92 microRNAs (type 2). Since miR-17-92 expression is transcriptionally regulated by MYC transcription factors, it has been postulated that Feingold syndrome type 1 and 2 may be caused by a common molecular mechanism. Here we show that Mir17-92 deficiency upregulates TGF-β signaling, whereas Mycn -deficiency downregulates PI3K signaling in limb mesenchymal cells. Genetic or pharmacological inhibition of TGF-β signaling efficiently rescues the skeletal defects caused by Mir17-92 deficiency, suggesting that upregulation of TGF-β signaling is responsible for the skeletal defect of Feingold syndrome type 2. By contrast, the skeletal phenotype of Mycn -deficiency is partially rescued by Pten heterozygosity, but not by TGF-β inhibition. These results strongly suggest that despite the phenotypical similarity, distinct molecular mechanisms underlie the pathoetiology for Feingold syndrome type 1 and 2. Heterozygous mutations in MYCN or MIR17HG in humans cause Feingold syndrome that is characterized by skeletal developmental defects including microcephaly, short stature, and brachysyndactyly with diminished middle phalanxes [1] , [2] , [3] . MYCN , a member of the MYC family proto-oncogenes, encodes a transcription factor that regulates genes that promote cell growth and proliferation [4] . Previous studies have shown that MYC (Myc in mice) transcription factors bind directly to the MIR17HG gene ( Mirc1 , also known as Mir17-92 in mice) to stimulate the expression of miR-17-92 microRNAs (miRNAs) encoded by this gene [5] , [6] . miR-17-92 cluster miRNAs are oncogenic miRNAs that have been studied mainly in the context of cancers [7] , [8] . miR-17-92 miRNAs regulate genes involved in cell cycle and apoptosis, such as Bim (Bcll11) [9] , [10] and E2f1 [5] , as well as target genes encoding signaling molecules [9] , [11] , [12] , [13] in a context-dependent manner to promote tumorigenesis. miR-17-92 miRNA family miRNAs, comprised of four functionally overlapping groups of miRNAs, are also encoded by two additional paralogous genes, MIR106B ( Mirc3 , also known as Mir106b-25 in mice) and MIR106A ( Mirc2 , also known as Mir106a-363 in mice). The physiologic role of miR-17-92 family miRNAs during animal development was demonstrated by genetic mutant mice missing these genes [10] . Homozygous deletion of Mir17-92 in mice impairs animal growth and causes prenatal lethality. Additional deletion of Mir106b-25 results in significantly more severe developmental defects, providing genetic evidence for the overlapping function of these genes. Based on the fact that deletion of either MYCN or Mir17HG results in similar skeletal defects in humans and that miR-17-92 expression is regulated by Myc transcription factors, it has been hypothesized that Mycn and miR-17-92 miRNAs function in the same pathway to regulate skeletal development [2] . To test this hypothesis, we conditionally deleted Mir17-92 with or without deletion of Mir106b-25 in the developing limb bud and skull mesenchyme. In this study, we present evidence that Mycn and miR-17-92 miRNAs regulate skeletal progenitor cell proliferation through distinct signaling pathways. We show that overactivation of TGF-β signaling causes the skeletal defects of miR-17-92 miRNA-deficient limbs and the skull, whereas downregulation of PI3K/Akt signaling is a major contributor to the skeletal phenotype caused by Mycn- deficiency. This study using in vivo models also suggests that physiological effects of miRNAs and transcription factors, which regulate multiple genes, converge onto relatively limited signaling pathways. Generation of mouse models of Feingold syndrome patients In order to determine physiologic roles of miR-17-92 miRNAs in skeletal development, we deleted Mir17-92 with or without its paralogous gene, Mir106b-25 , in skeletal mesenchymal cells using Prx1-Cre transgenic mice and floxed Mir17-92 and Mir106b-25 -null mice. Mice with heterozygous Mir17-92 deletion ( Prx1-Cre:Mir17-92 fl/+ ) exhibited modest skeletal defects similar to those in germline heterozygous null mice [2] (Supplementary Fig. 1a-d). The skeletal phenotype was more pronounced after deletion of both alleles of Mir17-92 (Fig. 1 ; Supplementary Fig. 1a-d). Simultaneous deletion of Mir17-92 and Mir106b-25 (doubly conditional knockout, Prx1-Cre:Mir17-92 fl/fl :Mir106b-25 − /− , 17 dKO) caused microcephaly, cutaneous syndactyly, and brachydactyly, phenotypes similar to those observed in patients with Feingold syndrome type 2 (Fig. 1a–d ). While heterozygous Mycn germline deletion in mice does not cause detectable skeletal abnormalities [14] , conditional deletion of Mycn in developing limbs ( Prx1-Cre:Mycn fl/fl , Mycn cKO) resulted in severe brachysyndactyly similar to that observed in patients with Feingold syndrome type 1 and also in mice previously reported [15] (Fig. 1a–d ). Fig. 1 Generation of mouse models of Feingold syndrome. a Forelimbs of wildtype control (Ctrl), Mycn Knockout ( Prx1-Cre:Mycn fl/fl , Mycn cKO), Mir17-92 knockout ( Prx1-Cre:Mir17-92 fl/fl , 17 KO), and Mir17-92 and Mir106b-25 doubly conditional knockout ( Prx1-Cre:Mir17-92 fl/fl :Mir106b-25 −/− , 17 dKO) mice at postnatal day (P) 16. 17 KO mutants exhibit mild brachydactyly in the fifth digit (double-headed arrows). Cutaneous syndactyly (arrows) and severe brachydactyly are presented in 17 dKO and Mycn cKO mice. Scale bar, 0.5 cm. b Alizarin red and alcian blue staining of the forelimb and magnified views of the fifth digit of corresponding mice in a . 17 KO mutants show shortening of the middle phalanx (M) (brackets) of the fifth digit. 17 dKO and Mycn cKO mutants show severe brachymesophalangy and the absence of the middle phalanx of the fifth digit (arrows). c Alizarin red and alcian blue staining of the skull of corresponding mice in a . Mycn cKO, 1 7 KO, and 17 dKO mice show microcephaly and a frontal bone ossification defect (arrows). Scale bar, 1 cm. d Quantification of the length of the fifth M and fifth metacarpal bone (5th MC) and the ratio of 5th M to 5th MC. Values are expressed as mean ± SE ( n = 5 in each group, * p < 0.001 vs. Ctrl). ND, not detected. e Relative expression of five miRNAs encoded in the Mir17-92 gene in limb bud mesenchymal cells isolated from Mycn cKO embryos at embryonic day 14.5. (relative to control littermate samples, n = 5 each group, *<0.001 vs. Ctrl at every time point). f Hindlimbs of wildtype Ctrl, Mycn cKO, and Mycn Knockout overexpressing Mir17-92 ( Prx1-Cre:Mycn fl/fl :Mir17-92 Tg , Mycn cKO: 17 Tg) (upper panels) and alizarin red and alcian blue staining of the hindlimbs of corresponding genotypes (bottom panels). Mir17-92 overexpression partially rescues the skeletal defects of Mycn cKO mutants. Cutaneous syndactyly (white arrows) and shortening of the fifth digit in Mycn cKO mutants are rescued by overexpression of Mir17-92 whereas fused fourth and fifth metatarsal bones still remain (bottom panels). Scale bar, 0.5 cm Full size image Mycn- deficient limb mesenchymal cells isolated from embryos at indicated embryonic days (E) showed significant reductions in miR-17-92 miRNA levels over time, as assessed by quantitative RT-PCR (qRT-PCR) and in situ hybridization (Fig. 1e ; Supplementary Fig. 2 ). Thus, we attempted to rescue the skeletal phenotype of Mycn -deficient limbs by overexpressing miR-17-92 miRNAs using Cre-inducible Mir17-92 transgenic mice [9] . Mir17-92 overexpression in transgenic mice ( Prx1-Cre:Mir17-92 Tg , 17 Tg) caused limb overgrowth (Supplementary Fig. 3 ), and it partially rescued the skeletal abnormalities of Mycn cKO mice (Fig. 1f ). These results are consistent with the notion that the action of Mycn is mediated, at least in part, by miR-17-92 miRNAs in skeletal development. Proliferation defects in miR-17-92 miRNA-deficient cells To assess the biological consequence of loss of Mir17-92 and Mir106b-25 in the skeletal mesenchyme, we measured cell proliferation and apoptosis in the skull and limbs of mutant embryos. Simultaneous loss of Mir17-92 and Mir106b-25 in the early limb bud and skull mesenchyme caused a significant decrease in cell proliferation (Fig. 2a–c ), which was also confirmed in vitro (Fig. 2d ). We did not find significant changes in cell death assessed by the TUNEL assay (Supplementary Fig. 4a ). The domain expressing Sox9 , a marker of precartilaginous condensations, was reduced in size in 17 dKO mice at E9.5 and E11.5, presumably due to the proliferation defect of 17 dKO limb mesenchymal cells (Fig. 2e ). 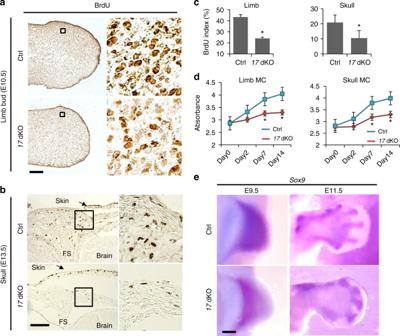Fig. 2 Proliferation defect in cells missingMir17-92andMir106b-25.a–dLoss ofMir17-92andMir106b-25(17dKO) impairs skeletal mesenchymal cell proliferation. SinceMir106b-25-null mice show no skeletal abnormalities,Mir106b-null mice were used as the control.aBrdU labeling on limb bud sections ofMir17-92fl/fl:Mir106b-25−/−(Ctrl) andPrx1-Cre:Mir17-92fl/fl:Mir106b-25−/−(17dKO) embryos at embryonic day (E) 10.5.bBrdU labeling of coronal skull sections of Ctrl and17dKO embryos at E13.5.cThe BrdU-positive cells were significantly reduced in the17dKO limb bud and skull mesenchyme (n= 6, *p< 0.05).dCell proliferation assay on limb bud and skull mesenchymal cells (MC) in vitro. Primary mesenchymal fibroblasts isolated fromMir17-92fl/fl:Mir106b-25−/−embryos were transduced with adenoviruses expressing a Cre recombinase (17dKO) or a yellow fluorescent protein (Ctrl) to deleteMir17-92in vitro. The efficient reduction (85 ± 5%) in miR-17-92 miRNAs was confirmed by qRT-PCR.Mir17-92-deficient limb bud and calvarial mesenchymal cells showed significantly impaired proliferation over time compared with control, as assessed by an index of the increase in cell mass (n= 5, *p< 0.05).eWhole-mount in situ hybridization forSox9shows a reduction in size of theSox9-positive domain at E9.5 and E11.5. FS frontal suture. Scale bar, 100 μm Conditional deletion of Mir17-92 and Mir106b-25 exclusively in the cells of the precartilaginous condensation and their descendants using Col2a1-Cre transgenic mice caused no obvious skeletal abnormalities (Supplementary Fig. 4b ), suggesting that the proliferation defect in cells of the limb bud mesenchyme, but not cells in the precartilaginous condensation, is responsible for the skeletal abnormalities of 17 dKO mice. Since Mycn deficiency also reduces limb bud cell proliferation [15] , these findings suggest that similar cellular mechanisms underlie the pathogenesis of Feingold syndrome type 1 and type 2. Fig. 2 Proliferation defect in cells missing Mir17-92 and Mir106b-25 . a – d Loss of Mir17-92 and Mir106b-25 ( 17 dKO) impairs skeletal mesenchymal cell proliferation. Since Mir106b-25 -null mice show no skeletal abnormalities, Mir106b- null mice were used as the control. a BrdU labeling on limb bud sections of Mir17-92 fl/fl :Mir106b-25 − / − (Ctrl) and Prx1-Cre:Mir17-92 fl/fl :Mir106b-25 − /− ( 17 dKO) embryos at embryonic day (E) 10.5. b BrdU labeling of coronal skull sections of Ctrl and 17 dKO embryos at E13.5. c The BrdU-positive cells were significantly reduced in the 17 dKO limb bud and skull mesenchyme ( n = 6, * p < 0.05). d Cell proliferation assay on limb bud and skull mesenchymal cells (MC) in vitro. Primary mesenchymal fibroblasts isolated from Mir17-92 fl/fl :Mir106b-25 −/ − embryos were transduced with adenoviruses expressing a Cre recombinase ( 17 dKO) or a yellow fluorescent protein (Ctrl) to delete Mir17-92 in vitro. The efficient reduction (85 ± 5%) in miR-17-92 miRNAs was confirmed by qRT-PCR. Mir17-92 -deficient limb bud and calvarial mesenchymal cells showed significantly impaired proliferation over time compared with control, as assessed by an index of the increase in cell mass ( n = 5, * p < 0.05). e Whole-mount in situ hybridization for Sox9 shows a reduction in size of the Sox9 -positive domain at E9.5 and E11.5. FS frontal suture. Scale bar, 100 μm Full size image TGF-β and STAT3 signaling upregulation in Mir17-92 -deficiency Although a miRNA potentially regulates hundreds of target genes, it is proposed that miRNA–RNA interactions are evolutionarily selected to cooperatively regulate certain biological pathways [16] , [17] , [18] . In addition to directly regulating genes involved in cell cycle and apoptosis [5] , [9] , miR-17-92 miRNAs are reported to regulate genes encoding signaling molecules in a context-dependent manner to promote tumorigenesis [11] , [13] , [19] . Therefore, we first determined the status of major signaling pathways in primary limb or skull mesenchymal cells missing Mir17-92 and Mir106b-25 . At the basal culture condition, we found upregulation in TGF-β and JAK/STAT3 signaling (Fig. 3a, b ). In addition, Mir17-92:Mir106b-25- deficient cells showed a greater response in Smad2 phosphorylation than control after acute stimulation with TGF-β1 (Fig. 3c ). The type II TGF-β receptor, Tgfbr2, a predicted target of miR-17 and miR-19 group miRNAs [19] , was upregulated at both the protein and mRNA levels (Fig. 3a, d ). Since loss of miR-17 group miRNAs (miR-17 and miR-20a) causes skeletal defects in mice [20] , we tested whether miR-17 can suppress gene expression via the predicted target sequence of Tgfbr2 by luciferase reporter assay. miR-17 co-transfection significantly reduced the expression of a luciferase reporter construct with the wildtype, but not with a mutated, binding sequence (Fig. 3e ). Although Bim and Pten were previously identified as critical miR-17-92 targets in lymphogenesis and tumorigenesis [9] , [10] , we did not find upregulation in Bim or Pten in 17 dKO mesenchymal cells (Fig. 3d ), supporting the notion that the regulatory role of miR-17-92 miRNAs is dependent on the cellular context. Fig. 3 TGF-β and STAT3 upregulation in miR-17-92 miRNA-deficient cells. a Immunoblot analysis on indicated proteins using protein lysates from cells cultured in DMEM containing 10% FBS. Levels of p-Smad2, Tgfbr2, and p-Stat3 (arrows) are increased in Mir17-92:Mir106b-25 -deficient limb bud cells ( 17 dKO). b Quantification of the p-Smad2 to total Smad2 (t-Smad2) and p-Stat3 to total Stat3 (t-Stat3) protein ratios based on western blot data ( n = 3, * p < 0.05). c Increased TGF-β signaling in 17 dKO cells upon stimulation. Serum-starved cells were treated with 50 ng/ml TGF-β1. Smad2 phosphorylation was analyzed at the indicated time points. 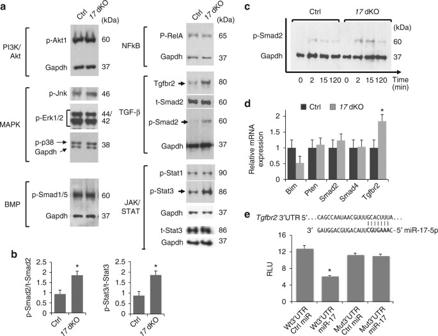Fig. 3 TGF-β and STAT3 upregulation in miR-17-92 miRNA-deficient cells.aImmunoblot analysis on indicated proteins using protein lysates from cells cultured in DMEM containing 10% FBS. Levels of p-Smad2, Tgfbr2, and p-Stat3 (arrows) are increased inMir17-92:Mir106b-25-deficient limb bud cells (17dKO).bQuantification of the p-Smad2 to total Smad2 (t-Smad2) and p-Stat3 to total Stat3 (t-Stat3) protein ratios based on western blot data (n= 3, *p< 0.05).cIncreased TGF-β signaling in17 dKOcells upon stimulation. Serum-starved cells were treated with 50 ng/ml TGF-β1. Smad2 phosphorylation was analyzed at the indicated time points.dRelative mRNA expression of known targets of miR-17-92 miRNAs in17 dKOlimb bud cells (n= 3, *p< 0.05).eLuciferase reporter assay for miR-17 regulation onTgfbr2binding site. Primary limb bud cells were co-transfected with control miRNA mimic (Ctrl miR) or mmu-miR-17-5p (miR-17) and a luciferase reporter construct carrying a wildtype (Wt 3′UTR) or mutated 3′UTR (Mut 3′UTR) sequence of mouseTgfbr2. The predicted binding sequence ofTgfbr23′UTR and relative luciferase units (RLU) are shown (n= 6, *p<0.001) d Relative mRNA expression of known targets of miR-17-92 miRNAs in 17 dKO limb bud cells ( n = 3, * p < 0.05). e Luciferase reporter assay for miR-17 regulation on Tgfbr2 binding site. Primary limb bud cells were co-transfected with control miRNA mimic (Ctrl miR) or mmu-miR-17-5p (miR-17) and a luciferase reporter construct carrying a wildtype (Wt 3′UTR) or mutated 3′UTR (Mut 3′UTR) sequence of mouse Tgfbr2 . The predicted binding sequence of Tgfbr2 3′UTR and relative luciferase units (RLU) are shown ( n = 6, * p < 0.001) Full size image Causal role of TGF-β signaling in cell proliferation defect To test whether the upregulation of the TGF-β or JAK/STAT3 signaling was responsible for the proliferation defect observed in 17 dKO cells, we inhibited these signaling pathways using pathway-specific inhibitors in vitro. Whereas treatment with the STAT3 inhibitor, S31-201, failed to promote proliferation of 17 dKO cells in vitro (Fig. 4a, b ), treatment with the TGF-β receptor inhibitor, LY364947, significantly ameliorated the proliferation defect of 17 dKO cells (Fig. 4c, d ). This finding was confirmed by experiments using GW788388, another TGF-β receptor inhibitor, and also using the neutralizing antibody against TGF-β ligands, 1D11 (Supplementary Fig. 5a, b ). These results suggest that the TGF-β upregulation is responsible for the proliferation defect, a finding consistent with the previous reports that overactivation of TGF-β signaling reduces limb mesenchymal cell proliferation and inhibits limb growth [21] , [22] . Fig. 4 Rescue of cell proliferation defects with TGF-β receptor inhibitors. a Cell proliferation assay on control (Ctrl) and Mir17-92:Mir106b-25 -deficient ( 17 dKO) limb bud mesenchymal cells treated with vehicle (DMSO) or a STAT3 inhibitor (STAT3 inh, S31-201, 100 µM). Ctrl and 17 dKO limb bud cells were prepared by transducing YPF (Ctrl) or Cre ( 17 dKO) in vitro. STAT3 inhibitor treatment shows no significant improvement in 17 dKO cell proliferation. b Treatment of limb bud cells with S31-201 downregulates the p-Stat3 level; *non-specific band. c Cell proliferation assay on Ctrl and 17 dKO (dKO) cells treated with DMSO or a TGF-β receptor inhibitor (Tgfbr inh, Ly364947, 0.2 µM). Treatment with Ly364947 has no significant effect on control cells whereas it significantly ameliorates the proliferation defect of 17 dKO cells ( n = 6, * p < 0.05 vs. 17 dKO + DMSO). d Treatment of limb bud cells with Ly364947 downregulates the p-Smad2 level. e – g Ly364947 treatment efficiently rescues the skeletal defects of 17 dKO mutants. Ly364947 (1 mg/kg/day, i.p.) was injected into pregnant and nursing mothers from E9.5 through P7.5, and then injected directly into individual mice. The shortening of the fifth digit (double arrows) syndactyly (white arrows) ( e ), missing middle phalanx (M) ( f ), and microcephaly and frontal bone ossification defect (black arrows) ( g ) in 17 dKO mutants were ameliorated by Ly364947 treatment. h Quantification of the length of the fifth mesophalanx (5th M), fifth metacarpal bone (5th MC), and the ratio of 5th M to 5th MC. Values are expressed as mean ± SE ( n = 6 each group, p < 0.001 vs. dKO). Scale bars: 0.5 cm in e , 1.0 cm in g . D distal phalanx; P proximal phalanx Full size image TGF-β inhibition rescues skeletal defects of 1 7 dKO mice We treated 17 dKO mice with TGF-β receptor inhibitors from E9.5 through postnatal day (P) 16.5. 17 dKO mice treated with LY364947 showed significant normalization of limb and skull development (Fig. 4e–h ). Moreover, genetic suppression of TGF-β signaling via conditionally deleting one allele of Tgfbr2 in 17 dKO mice ( 17 dKO :Tgfbr2 Het) also partially rescued the skeletal abnormalities of 17 dKO mice (Supplementary Fig. 5c ). A short-term treatment regimen during early stages of limb development (E9.5–E15.5) with TGF-β receptor inhibitor mostly rescued the limb and skull abnormalities whereas treatment during late embryonic stages (E15.5–E18.5) showed no effect (Supplementary Fig. 5d ). These data suggest that miR-17-92 miRNA-mediated suppression of TGF-β signaling through Tgfbr2 downregulation is particularly important during early stages of skeletal development and that the TGF-β signaling upregulation is responsible for skeletal defects in Feingold syndrome type 2. TGF-β inhibitor treatment also rescued the digit phenotype of mice with heterozygous Mir17-92 deletion, a genetic alteration close to that of patients with Feingold syndrome type 2, further supporting this notion (Supplementary Fig. 6a ). Distinct molecular mechanisms in 17 dKO and Mycn cKO mice In contrast to 17 dKO mice, suppression of TGF-β signaling via Tgfbr2 heterozygous deletion or TGF-β receptor inhibitor treatment failed to rescue the skeletal defects of Mycn cKO mice (Fig. 5a, b ; Supplementary Fig. 6b ). Consistent with this result, we did not find upregulation in TGF-β signaling in Mycn -deficient cells, as indicated by the unaltered level of p-Smad2 (Fig. 5c, d ). These results conflict with the previously proposed model in which miR-17-92 miRNAs mediate Mycn’s action [2] , and are also inconsistent with our earlier observations that miR-17-92 expression is reduced in E14.5 Mycn -deficient limbs and that miR-17-92 overexpression rescues the Mycn cKO digit phenotype (Fig. 1e, f ). However, we noted that the reduction of miR-17-92 miRNA expression levels in Mycn cKO cells was relatively modest at E10.5 when TGF-β suppression by miR-17-92 miRNAs is critical to maintain limb mesenchymal cell proliferation (Fig. 1e ). Consistent with this finding, known miR-17-92 miRNAs target genes, including Tgfbr2 , were not deregulated in Mycn -deficient cells at E10.5 (Fig. 5d ). We compared the gene expression profiles of Mycn -deficient and 17 dKO limb mesenchymal cells by RNA-Seq, but found an only limited overlap in genes whose expression was altered in these two groups (Supplementary Fig. 7a ; Supplementary Data 1 ). Together, these data demonstrate that, unlike in the model of Feingold syndrome type 2, TGF-β deregulation does not play a causal role in the pathogenesis of the type 1 Feingold syndrome model ( Mycn deletion). Fig. 5 Distinct mechanisms in Feingold syndrome mouse models. a Forelimbs of mice with indicated genotypes at postnatal day 16. Wildtype control (Ctrl), Mycn conditional Knockout ( Prx1-Cre:Mycn fl/fl , Mycn cKO), Mycn cKO in which one allele of Tgfbr2 is deleted ( Prx1-Cre:Mycn fl/fl :Tgfbr2 fl/+ , Mycn cKO :Tgfbr2 Het), Mir17-92 and Mir106b-25 doubly conditional knockout ( Prx1-Cre:Mir17-92 fl/fl :Mir106b-25 − / − , 17 dKO), and 17 dKO in which one allele of Tgfbr2 is deleted ( Prx1-Cre:Mir17-92 fl/fl :Mir106b-25 −/− :Tgfbr2 fl/+ , 17 dKO: Tgfbr2 Het). Unlike 17 dKO mice, the digit abnormalities of Mycn cKO mutants are not rescued by Tgfbr2 heterozygous deletion. b Alizarin red and alcian blue staining of forelimbs of corresponding mice in a . Scale bars, 0.5 cm. More than three rescued mice per each model were analyzed to confirm the reproducibility. c Immunoblot analysis for indicated proteins upon treatment with 10% fetal bovine serum (FBS) at indicated time points (top panel). Primary mesenchymal fibroblasts from limb buds of E10.5 Mycn fl/fl embryos were transduced with adenoviruses expressing a Cre recombinase (KO) or a yellow fluorescent protein (Ctrl) to delete Mycn in vitro. Cells were serum starved for 1 h before stimulation. The efficient reduction in the Mycn protein level was confirmed. Levels of p-Akt (Thr308) and p-S6k are decreased in Mycn -deficient limb bud cells (KO). Quantification of p-Akt relative to total Akt (t-Akt) and p-Smad2 to total Smad2 (t-Smad2) at time 0 based on the western blot data (bottom panels) ( n = 3, * p < 0.05). d Relative expression of previously reported targets of miR-17-92 miRNAs in Mycn cKO limb bud mesenchymal cells isolated from embryos at age E10.5. Y axis, arbitrary units Full size image Role of PI3K downregulation in Mycn cKO mice To further investigate the molecular mechanism for the type 1 model, we revisited the fact that miR-17-92 overexpression rescued the Mycn cKO digit phenotype. The miR-17-92 miRNA levels in the limb mesenchymal cells of 17 Tg mice were four times more abundant than those in control (Supplementary Fig. 8a ). We also found that these supraphysiological levels of miR-17-92 miRNAs suppressed the expression of Pten , a negative regulator of phosphoinositide 3-kinase (PI3K)/Akt signaling, and upregulated the phospho-Akt (p-Akt) level (Supplementary Fig. 8b, c ). Thus, we hypothesized that deregulation of the PI3K/Akt signaling pathway was involved in the pathogenesis of the Mycn cKO phenotype. Indeed, we found that Mycn -deficient mesenchymal cells showed a decreased level of p-Akt (Thr308), suggesting downregulation of the PI3K signaling pathway (Fig. 5c ). To test whether the suppression of the PI3K signaling pathway is responsible for the skeletal abnormalities in Mycn cKO, we deleted one allele of Pten in Mycn cKO mice ( Mycn cKO :Pten Het). Although Pten haploinsufficiency itself did not cause any skeletal phenotype, we found that Pten heterozygous deletion in Mycn -deficient skeletal progenitor cells partially rescued the skeletal abnormality of Mycn cKO mice to a similar extent to Mir17-92 overexpression ( Mycn cKO: 17 Tg) (Fig. 6a, b ). We confirmed that the p-Akt level increased in Mycn cKO limb bud cells after deletion of one allele of Pten (Fig. 6c ). In contrast, Pten heterozygous deletion showed no effect on the 17 dKO skeletal phenotype (Supplementary Fig. 8d ). These data suggest that downregulation of the PI3K signaling pathway plays a major pathogenic role in the Feingold syndrome type 1, but not type 2. Fig. 6 PI3K downregulation contributes to the Mycn cKO phenotype. a Hindlimbs of mice with indicated genotypes at postnatal day 16. Wildtype control (Ctrl), heterozygous Pten mutant ( Prx1-Cre:Pten fl/+ , Pten Het), Mycn Knockout ( Prx1-Cre:Mycn fl/fl , Mycn cKO), Mycn cKO in which one allele of Pten is deleted ( Prx1-Cre:Mycn fl/fl :Pten fl/+ , Mycn cKO :Pten Het), and Mycn Knockout overexpressing Mir17-92 ( Prx1-Cre:Mycn fl/fl :Mir17-92 Tg , Mycn cKO :17 Tg). Pten heterozygous deletion partially rescues the skeletal abnormalities of Mycn cKO mutants. Cutaneous syndactyly and brachydactyly are partially rescued, while the fused metatarsals and shortening of mid phalanxes remain. The fifth metacarpal bones, subjected to measurement in b , are indicated by brackets. Scale bars, 0.5 cm. b Quantification of the length (µm) of fifth metacarpal bones of mice with indicated genotypes ( n = 6 for Ctrl and Mycn cKO, n = 5 for Pten Het and Mycn cKO :Pten Het , n = 4 for Mycn cKO :17 Tg; * p < 0.01 vs. Ctrl, ** p < 0.01 vs. Mycn cKO). c PI3K signaling was assessed by p-Akt (Thr308) in limb bud cells isolated from E 10.5 mice with indicated genotype. d Immunoblot analysis for phospho-Pten (p-Pten) and total Pten (t-Pten) isolated from Mycn cKO and wildtype littermate limb bud cells. The p-Pten level is decreased in Mycn -deficient skeletal progenitor cells whereas the t-Pten level is unchanged. e Immunoblot analysis for casein kinase 2 beta phosphorylation on S209 (p-CK2) in limb bud mesenchymal cells isolated from E10.5 Mycn cKO and wildtype littermates. p-CK2 is decreased in Mycn -deficient cells; *non-specific band. f Proposed model. Upregulation of TGF-β signaling plays a causal role in the skeletal defect of Feingold syndrome type 2 ( Mir17-92 mutation), whereas downregulation of the PI3K signaling plays a major pathophysiologic role in Feingold syndrome type 1 ( Mycn mutation). Mycn partially regulates miR-17-92 miRNA levels, but the contribution of this regulation in limb development is limited (dotted arrow). Overexpression of miR-17-92 miRNAs can suppress Pten, although miR-17-92 miRNAs have limited regulatory effects on Pten expression at the physiological level (dotted inhibitory line) Full size image Regarding the mechanism by which Mycn deficiency reduces PI3K signaling, there were no significant changes in the expression level of genes related to the PI3K complex, Pten , or their downstream effectors in Mycn cKO limb bud cells (Supplementary Fig. 7b ). However, we found decreased phosphorylation of the tail region of Pten (p-Pten) that negatively regulates Pten activity [23] (Fig. 6d ). 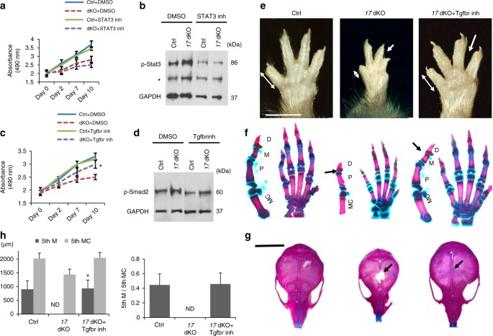Fig. 4 Rescue of cell proliferation defects with TGF-β receptor inhibitors.aCell proliferation assay on control (Ctrl) andMir17-92:Mir106b-25-deficient (17dKO) limb bud mesenchymal cells treated with vehicle (DMSO) or a STAT3 inhibitor (STAT3 inh, S31-201, 100 µM). Ctrl and17dKO limb bud cells were prepared by transducing YPF (Ctrl) or Cre (17dKO) in vitro. STAT3 inhibitor treatment shows no significant improvement in17dKO cell proliferation.bTreatment of limb bud cells with S31-201 downregulates the p-Stat3 level; *non-specific band.cCell proliferation assay on Ctrl and17dKO (dKO) cells treated with DMSO or a TGF-β receptor inhibitor (Tgfbr inh, Ly364947, 0.2 µM). Treatment with Ly364947 has no significant effect on control cells whereas it significantly ameliorates the proliferation defect of17dKO cells (n= 6, *p<0.05 vs.17dKO + DMSO).dTreatment of limb bud cells with Ly364947 downregulates the p-Smad2 level.e–gLy364947 treatment efficiently rescues the skeletal defects of17dKO mutants. Ly364947 (1 mg/kg/day, i.p.) was injected into pregnant and nursing mothers from E9.5 through P7.5, and then injected directly into individual mice. The shortening of the fifth digit (double arrows) syndactyly (white arrows) (e), missing middle phalanx (M) (f), and microcephaly and frontal bone ossification defect (black arrows) (g) in17dKO mutants were ameliorated by Ly364947 treatment.hQuantification of the length of the fifth mesophalanx (5th M), fifth metacarpal bone (5th MC), and the ratio of 5th M to 5th MC. Values are expressed as mean ± SE (n= 6 each group,p< 0.001 vs. dKO). Scale bars: 0.5 cm ine, 1.0 cm ing. D distal phalanx; P proximal phalanx Casein kinase 2 (CK2) is a major regulator of Pten phosphorylation and activity [24] , [25] , [26] , and CK2 and Myc have been shown to synergistically promote oncogenesis via the CK2’s promoting action on Myc stabilization [27] . Therefore, we examined the expression and activation of CK2. While the total expression level of CK2 genes was unaltered (Supplementary Fig. 7c, d ), CK2 phosphorylation, which reflects CK2 activity [28] , was reduced in Mycn -deficient cells (Fig. 6e ). These results suggest that the downregulation of the CK2/Pten cascade is responsible, at least in part, for the reduced PI3K signaling caused by Mycn deficiency. In this study, we generated mouse models that exhibited skeletal phenotypes similar to those in patients with Feingold syndrome type 1 and type 2 by conditionally deleting Mycn and Mir17-92 , respectively, in skeletal progenitors. Our findings strongly suggest that TGF-β signaling upregulation in mesenchymal progenitor cells plays a major causal role in the skeletal abnormalities of Feingold syndrome type 2, whereas downregulation of the PI3K signaling pathway significantly contributes to the pathogenesis of Feingold syndrome type 1 (Fig. 6f ). Although these mouse models are not exact genetic equivalents of human patients with heterozygous deletions of these genes, considering that heterozygous germline-null mice do not fully recapitulate the phenotypes of patients with Feingold syndrome type 1 and type 2 and that our mouse models recapitulate well the skeletal abnormalities of patients, our mouse models likely share the same pathophysiological mechanisms of these diseases in humans. In addition, the finding that TGF-β inhibition was able to rescue the digit defect (shortening of the middle phalanx) of heterozygous Mir17-92 conditional deletion also supports that the TGF-β deregulation underlies the pathogenesis of Feingold syndrome type 2. Considering that the cellular mechanism that accounts for the skeletal defects, i.e., reduced proliferation of mesenchymal progenitors, appears to be common in Mir17-92:106b-25 -deficient (present study) and Mycn -deficient limbs and skulls [15] and that the well-established molecular relationship between Myc transcription factors and miR-17-92 miRNAs, our finding that deficiencies of Mycn and miR-17-92 miRNAs causes aberrations in distinct signaling pathways was unexpected. As previous study showed [2] , we also found partial reductions in miR-17-92 miRNAs in Mycn -deficient limbs. Considering that Mycn -deficient limbs show a skeletal phenotype more severe than that of Mir17-92:106b-25 doubly conditional nullizygotes, the partial reduction of miR17-92 miRNAs in Mycn -deficient limbs may have only limited biological effects. In the mouse model for Feingold syndrome type 2, using genetic and pharmacological interventions, we have demonstrated that the upregulation in TGF-β signaling due to derepression of Tgfbr2 , a direct target of multiple miR-17-92 miRNAs, plays the causal role. The fact that suppression of TGF-β alone was able to almost completely rescue the skeletal defects of Mir-17-92:106b-25- deficient limbs and skulls indicates that Tgfbr2 is the most physiologically important target of miR-17-92 miRNAs in the context of skeletal development, despite the fact that miR-17-92 miRNAs regulates many other genes in diverse types of cells [29] . Deletion of the endogenous miR-17-92 miRNAs showed no effects on the expression of other known targets, including Pten. However, overexpression of miR-17-92 miRNAs to a supraphysiological level did suppress Pten. This result suggests that suppressive effects of miR-17-92 miRNAs on their targets are dependent on the cellular context, absolute expression level of miRNAs, and perhaps miRNA-target RNA stoichiometry. We have shown that the downregulation of PI3K/Akt signaling contributes to the skeletal phenotype of Mycn cKO mice. Myc transcription factors control cell growth and proliferation downstream of diverse signaling stimuli [30] ; however, little is known how Myc transcription factors regulate signaling pathways. We have found that Mycn -deficiency decreases Pten phosphorylation and CK2 activation, suggesting the alteration of the CK2/Pten pathway is likely the cause for the reduced PI3K/Akt signaling in Mycn- deficient cells. The precise mechanism by which Mycn deficiency alters the CK2/Pten pathway is unclear at the moment. In summary, we have demonstrated that distinct molecular mechanisms are responsible for skeletal phenotypes of mouse models of Feingold syndrome type 1 and type 2. Our results also suggest that targeting specific signaling pathways is a valid therapeutic approach to Feingold syndrome. Mice Floxed Mir17-92 mice and Mir106b-25 -null mice [10] , Cre-inducible CAG-Mir17-92 transgenic mice [9] , Prx1Cre transgenic mice [31] , Col2Cre transgenic mice [32] , and floxed Mycn mice [33] were previously described. Mice are in a C57/B6-dominant mixed background. Mutant mice were compared with littermate control mice except mice treated with chemical inhibitors during pregnancy. Since both males and females show the same phenotype with similar degrees, males and females were not discriminated. The mutant mice generally showed qualitative phenotypes; more than three independent experiments were performed to ensure the reproducibility. Due to the nature of experiments, no randomization or blinding was used. The animal experiments were approved by the Institutional Animal Care and Use Committee (IACUC) of the Massachusetts General Hospital and performed in accordance with the regulations and guidelines. Reagents Recombinant mouse TGF-β1 (#5231) was purchased from Cell Signaling Technology. Ly364947 (#S2805), GW788388 (#S2750), and S3I-201 (#S1155) were purchased from Selleck Chemicals. TGF-β receptor inhibitor injection TGF-β receptor inhibitors, Ly364947 and GW788388, were dissolved in DMSO at the concentration of 1 mg/ml and 2 mg/ml, respectively. Ly364947 (1 mg/kg/day) and GW788388 (1 mg/kg/day) were injected intraperitoneally (i.p.) into pregnant mothers or nursing mothers until P7.5. Mice older than P7.5 were individually injected. Skeletal preparation and histology Alizarin red and alcian blue staining was performed using a modified McLeod’s method [34] . For histological analysis, the embryos were dissected, fixed in 10% formalin, paraffin-processed, cut, and subjected to BrdU staining and TUNEL staining using the In situ Cell Death Detection kit (Sigma-Aldrich). Cell proliferation assays For BrdU labeling, BrdU (50 mg/kg) was injected into pregnant mice i.p. 2 h before euthanasia. BrdU was detected using the BrdU in situ staining kit (Invitrogen). The BrdU labeling index was calculated as the ratio of BrdU-positive stained nuclei over total nuclei. In vitro cell proliferation was quantified using the PrestoBlue Cell Viability Reagent (Molecular Probes) according to the manufacturer’s instruction. Primary limb bud cells isolation and culture Isolation and culture of primary limb bud cells of E9.5 through E11.5 mice were performed as previously described [35] . Briefly, embryos were isolated from timed-mated females by cesarean section. Limb buds, dissected using fine tweezers, were treated with 0.25% trypsin containing 2.21 mM EDTA for 5 min to disperse cells before plating. After overnight culture, cells were trypsinized and replated at the concentration of 5 × 10 5 /ml in a DMEM medium containing 10% fetal bovine serum (FBS). Upon reaching confluence, cells were collected to assess the basal status of indicated signaling pathways. Cells were also serum-starved for 3 h before stimulating with 10% FBS containing 50 ng/ml of TGF-β1. To assess Smad2 phosphorylation, cells were lysed at indicated time points and subjected to Western blot analysis. For RNA isolation, four limb buds of E10.5 and E11.5 embryos were directly lysed in Trizol. For E14.5 limbs, paws of four limbs were dissected to remove the skin and lysed in Trizol. For in vitro Mir17-92 deletion, primary limb cells isolated from Mir17-92 homozygous floxed, Mir106b null embryos at E10.5 and were cultured in a DMEM medium containing 10% FBS until reaching 50% confluence. Adenoviruses expressing either Cre or YFP (control) were then added to delete Mir17-92 . Then cells were split and grown in 96-well plates for indicated days. In situ hybridization Non-radioactive whole-mount in situ hybridization of mouse embryos was done using a standard protocol [36] . The Sox9 probe was previously described [37] . Section in situ hybridization for miR-17-5p was performed according to the standard protocol with minor modifications [38] . E14.5 forelimbs of Prx1-Cre:Mycn fl/fl mice and Cre -negative littermate control were formalin-fixed, paraffin-processed, cut at 5 µm thickness. The DIG-labeled miR-17 oligo probe (mmu-miR-17-5p; YD00615470-BCG) was purchased from Qiagen. Adenovirus production and infection Adenoviruses expressing Cre or YFP were gifts from Dr. Murat Bastepe (Harvard Medical School). Amounts of adenoviruses used for infection were empirically determined to achieve >75% infection efficiency. The infection efficiency was determined 2 days after infection by visualizing YFP for YFP-expressing adenoviruses or by quantifying floxed gene products for Cre-expressing adenoviruses. Primary embryonic limb bud cell isolation Prx1Cre: Mycn fl/+ male and Mycn fl/fl female mice were mated and mating was confirmed by the presence of a vaginal plug (considered as day 0.5 of gestation). Similarly, Prx1Cre: Mir17-92 fl/+ :Mir106b-25 +/− male and Mir17-92 fl/fl :Mir106b-25 − /− female mice were mated to generate doubly conditional knockout mice. On the day 10.5 of gestation, pregnant female mice were sacrificed. The uterus was removed and washed in sterile calcium and magnesium-free PBS. E10.5 embryos were then recovered from the uterus and washed several times in PBS. Distal parts of fore and hind limb buds of embryos were isolated under a dissecting microscope using two pairs of sharp forceps and lysed in TRIzol (Molecular Research Center, Cincinnati, OH, USA). Total RNA was extracted using the Direct-Zol TM RNA MiniPrep kit (Zymo Research, USA) according to the manufacturer’s instruction. RNA sequencing RNA-seq libraries were prepared with the Truseq mRNA kit (Illumina Inc., San Diego, CA, USA) with polyA + mRNA selection. Libraries were sequenced with the Illumina NextSeq system with 75 bp single end reads to generate 36–52 million reads per library. Reads were mapped to the mouse genome (mm10) with the STAR aligner [39] , and differential expression analyses between biologic groups were performed with edger [39] . The significance level was set at p < 0.05 (after correction for multiple hypothesis testing) for genes with mean FPKM >3 in at least one biologic group. qRT-PCR cDNA synthesis was performed using random hexamers using the DyNAmo cDNA Synthesis Kit (Finnzymes). Quantitative PCR was performed using the StepOnePlus Real-Time PCR System (Applied Biosystems) and the EvaGreen qRT-PCR mix (Solix BioDyne). Primer sequences are as follows: Pten-L, 5′-GAAAGGGACGGACTGGTGTA-3′ and Pten-R, 5′-AGTGCCACGGGTCTGTAATC-3′; GAPDH-L, 5′-CACAATTTCCATCCCAGACC-3′ and GAPDH-R, 5′-GTGGGTGCAGCGAACTTTAT-3′; Smad2-L, 5′-AGTATGGACACAGGCTCTCC-3′ and Smad2-R, 5′-GTCTGCCTTCGGTATTCTG-3′; Smad4-L, 5′-ATCTGAGTCTAATGCTACCAGC-3′ and Smad4-R, 5′-TTCTTTGATGCTCTGTCTTGG-3′; Bim-L, 5′-GCCCCTACCTCCCTACAGAC-3′ and Bim-R, 5′- GGCATCACCGTGGATATTTT-3′; Tgfbr2-L, 5′-GCAGTGGGAGAAGTAAAAGA-3′ and Tgfbr2-R, 5′- CCAGCCTGCCCCATAAGAGC-3′. Pik3r1-R, 5′-GCAGCTGAGTACCGAGAGAT-3′; Pik3r1-L, 5′-GCCACTCGTTCAGCTTCTTC-3′; Pik3r3-R, 5′-ACCGAGTACAAGCAGAGGAC-3′; Pik3r3-L, 5′-GCAAAGCCATATCCTCGAGC-3′; Pik3r5-R, 5′-TTTCAGGGAAGGTGGCTAGG-3′; Pik3r5-L, 5′-GTTCCGTGGCTTCTCTTCAC-3′; Pik3ip1-R, 5′-CAAAGAGGCACAGGTGTTCC-3′; Pik3ip1-L, 5′-TGTAGCCCACGATAATGCCA-3′; Akt1s1-R, 5′-AAGAGGACAGAAGCCCGATC-3′; Akt1s1-L, 5′-GGAAGTCGCTGGTATTGAGC-3′. Expression of miR-17-92 miRNAs and miR-106b-25 miRNAs were determined using the mirVana qRT-PCR miRNA Detection Kit (Ambion). Luciferase reporter assay A 350-bp-long DNA fragment containing the conserved miR-17 binding sequence (5′-GCACTTTA-3′) or a mutated sequence (5′-GC T CT A TA-3′) was PCR amplified using primers, Common R, 5′-GCAAGCTTCTCAGCTCCCTGGTCCATAA-3′ and Wt-F, 5′-GCACTAGTGATCAGCTAATTGACCAGATGCACTTTATTAATGCCTGTGTGTAAATACGAA-3′ or Mut-F, 5′-GCACTAGTGATCAGCTAATTGACCAGATGCTCTATATTAATGCCTGTGTGTAAATACGAA-3′ and subcloned into pMIR-REPORT miRNA Expression Reporter Vector System (AM5795, ThermoFisher) at the Hind III and Spe I sites. miR-17 miRIDIAN microRNA mimic and a control mimic were purchased from Dharmacon. 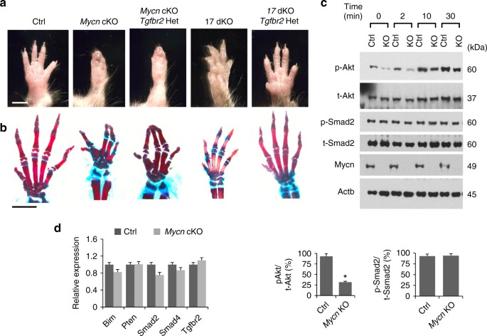Fig. 5 Distinct mechanisms in Feingold syndrome mouse models.aForelimbs of mice with indicated genotypes at postnatal day 16. Wildtype control (Ctrl),Mycnconditional Knockout (Prx1-Cre:Mycnfl/fl,MycncKO),MycncKO in which one allele ofTgfbr2is deleted (Prx1-Cre:Mycnfl/fl:Tgfbr2fl/+, MycncKO:Tgfbr2Het),Mir17-92andMir106b-25doubly conditional knockout (Prx1-Cre:Mir17-92fl/fl:Mir106b-25−/−,17dKO), and17dKO in which one allele ofTgfbr2is deleted (Prx1-Cre:Mir17-92fl/fl:Mir106b-25−/−:Tgfbr2fl/+,17dKO:Tgfbr2Het). Unlike17dKO mice, the digit abnormalities ofMycncKO mutants are not rescued byTgfbr2heterozygous deletion.bAlizarin red and alcian blue staining of forelimbs of corresponding mice ina. Scale bars, 0.5 cm. More than three rescued mice per each model were analyzed to confirm the reproducibility.cImmunoblot analysis for indicated proteins upon treatment with 10% fetal bovine serum (FBS) at indicated time points (top panel). Primary mesenchymal fibroblasts from limb buds of E10.5Mycnfl/flembryos were transduced with adenoviruses expressing a Cre recombinase (KO) or a yellow fluorescent protein (Ctrl) to deleteMycnin vitro. Cells were serum starved for 1 h before stimulation. The efficient reduction in the Mycn protein level was confirmed. Levels of p-Akt (Thr308) and p-S6k are decreased inMycn-deficient limb bud cells (KO). Quantification of p-Akt relative to total Akt (t-Akt) and p-Smad2 to total Smad2 (t-Smad2) at time 0 based on the western blot data (bottom panels) (n= 3, *p< 0.05).dRelative expression of previously reported targets of miR-17-92 miRNAs inMycncKO limb bud mesenchymal cells isolated from embryos at age E10.5.  Y axis, arbitrary units 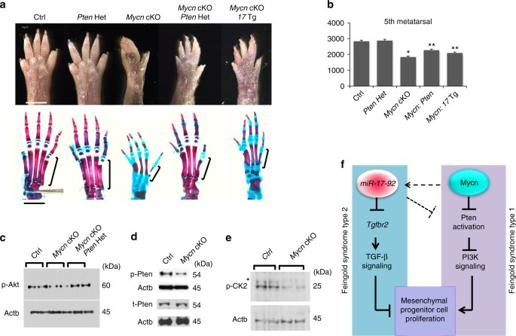Fig. 6 PI3K downregulation contributes to theMycncKO phenotype.aHindlimbs of mice with indicated genotypes at postnatal day 16. Wildtype control (Ctrl), heterozygousPtenmutant (Prx1-Cre:Ptenfl/+,PtenHet),MycnKnockout (Prx1-Cre:Mycnfl/fl,MycncKO),MycncKO in which one allele ofPtenis deleted (Prx1-Cre:Mycnfl/fl:Ptenfl/+, MycncKO:PtenHet), andMycnKnockout overexpressingMir17-92(Prx1-Cre:Mycnfl/fl:Mir17-92Tg, MycncKO:17Tg).Ptenheterozygous deletion partially rescues the skeletal abnormalities ofMycncKO mutants. Cutaneous syndactyly and brachydactyly are partially rescued, while the fused metatarsals and shortening of mid phalanxes remain. The fifth metacarpal bones, subjected to measurement inb, are indicated by brackets. Scale bars, 0.5 cm.bQuantification of the length (µm) of fifth metacarpal bones of mice with indicated genotypes (n= 6 for Ctrl andMycncKO,n= 5 forPten HetandMycncKO:Pten Het,n= 4 forMycncKO:17Tg; *p< 0.01 vs. Ctrl, **p< 0.01 vs.MycncKO).cPI3K signaling was assessed by p-Akt (Thr308) in limb bud cells isolated from E 10.5 mice with indicated genotype.dImmunoblot analysis for phospho-Pten (p-Pten) and total Pten (t-Pten) isolated fromMycncKO and wildtype littermate limb bud cells. The p-Pten level is decreased inMycn-deficient skeletal progenitor cells whereas the t-Pten level is unchanged.eImmunoblot analysis for casein kinase 2 beta phosphorylation on S209 (p-CK2) in limb bud mesenchymal cells isolated from E10.5MycncKO and wildtype littermates. p-CK2 is decreased inMycn-deficient cells; *non-specific band.fProposed model. Upregulation of TGF-β signaling plays a causal role in the skeletal defect of Feingold syndrome type 2 (Mir17-92mutation), whereas downregulation of the PI3K signaling plays a major pathophysiologic role in Feingold syndrome type 1 (Mycnmutation). Mycn partially regulates miR-17-92 miRNA levels, but the contribution of this regulation in limb development is limited (dotted arrow). Overexpression of miR-17-92 miRNAs can suppress Pten, although miR-17-92 miRNAs have limited regulatory effects on Pten expression at the physiological level (dotted inhibitory line) A renilla luciferase expression construct, a Tgfbr2 -UTR reporter construct, and the miR-17 mimic or control mimic were co-transfected to primary limb bud cells isolated from E12.5 embryos using Attractene transfection reagent (Qiagen) according to manufacturer’s instruction. Forty-eight hours after transfection, the cells were lysed, and luciferase and renilla luciferase activities were measured using the Dual-luciferase reporter assay system (Promega). Western blot analysis Anti-Smad2 (#5339), p-Smad2 (Ser465/467 #3108), p-Akt (Thr308, #2965), p-Akt (Ser473, #4060), NFkB (#3037), p-Erk (Ser259 #9911), p-p38 (#4511), p-Jnk (#4668), p-Stat3 (#9145), p-Stat1 (#9171), Tgfbr2 (#3713), p-IRS1 (Tyr895, 3070), p-Smad1/5(#9511), p-Pten (Ser380/Thr382/383, #9549), Pten (D4.3 #9188), and Act-b (13E5, #4970) antibodies were purchased from Cell Signaling Technology. Anti-p-Akt (T308) antibody (# 658320) was purchased from R&D Systems. Anti-Mycn (B8.4.B, #sc-53993) antibody was purchased from Santa Cruz Biotechnology. Anti-pCKIIβ (S209) antibody (STJ90892) was purchased from St Joh’s laboratory. Anti-Gapdh antibody (10R-2932) was purchased from Fitzgerald Industries International. Western blot analysis was performed according to the standard procedure. Uncropped blots are included in Supplemetary Figs. 9 – 12 . Data availability The RNA-seq data are uploaded to the ArrayExpress database with the accession number, E-MTAB-5671 ( https://www.ebi.ac.uk/arrayexpress/experiments/E-MTAB-5671/ ). Statistics Data are presented as mean ± SEM from indicated numbers of samples. For statistical analysis between the two groups, we used a 2-tailed Student’s t test; p values less than 0.05 were considered statistically significant. Sample numbers were determined based on the effect size obtained during preliminary experiments to obtain a power of 0.8.